Terminal supraparticle assemblies from similarly charged protein molecules and nanoparticles Self-assembly of proteins and inorganic nanoparticles into terminal assemblies makes possible a large family of uniformly sized hybrid colloids. These particles can be compared in terms of utility, versatility and multifunctionality to other known types of terminal assemblies. They are simple to make and offer theoretical tools for designing their structure and function. To demonstrate such assemblies, we combine cadmium telluride nanoparticles with cytochrome C protein and observe spontaneous formation of spherical supraparticles with a narrow size distribution. Such self-limiting behaviour originates from the competition between electrostatic repulsion and non-covalent attractive interactions. Experimental variation of supraparticle diameters for several assembly conditions matches predictions obtained in simulations. Similar to micelles, supraparticles can incorporate other biological components as exemplified by incorporation of nitrate reductase. Tight packing of nanoscale components enables effective charge and exciton transport in supraparticles and bionic combination of properties as demonstrated by enzymatic nitrate reduction initiated by light absorption in the nanoparticle. Self-organization of semiconductor or metal nanoparticles (NPs) leads to nano- and microscale superstructures with geometries reminiscent of those produced by biological macromolecules [1] , [2] , [3] , [4] , [5] , [6] , [7] . Distinct parallels can be also made between assemblies of globular proteins and those made by NPs [5] , [6] , [7] , [8] . While many geometrical motifs for assemblies of proteins are known, those between NP and biomacromolecules are limited. They are represented predominantly by extended assemblies, that is, those without defined size requirements for some assembly directions. Extended NP assemblies produce polydisperse nano- and microscale structures and can be exemplified by templated NP adsorbates [9] , cocrystallized NP–protein superlattices [7] and free-floating NP chains, sheets and ribbons of different lengths [1] , [3] , [10] . Whereas terminal assemblies are those that can be formed only with inherent size restrictions in all directions, for example, micelles, vesicles and viral capsids ( Supplementary Note 1 ). Such systems are fundamentally and technologically attractive due to their uniformity, versatility and simplicity of preparation. Terminal assemblies are not known for hybrid NP–biomacromolecule systems. Covalent bioconjugates [10] , [11] , electrostatic complexes between single-protein molecules and NPs [12] , [13] , biomolecular coronas around NPs [14] and similar structures [15] display dimensional restrictions, but it is difficult to classify them as terminal assemblies for reasons of preparative methods, small number of particles, uniformity or stability. Finding a way to make hybrid nano-bio terminal assemblies would open the door to a new diverse family of colloids. Besides being a potential analytical [13] and drug delivery tool [16] , the scientific value of such systems will be the possibility to integrate biological functions of proteins with optical and electrical properties of metallic and semiconducting materials. They may also uncover unknown biological effects of NPs present in the environment [17] . In this paper, we present a new type of protein–NP hybrid structures, known as supraparticles (SPs) [18] , that spontaneously assemble under a variety of conditions from cadmium telluride (CdTe) NPs and cytochrome C (CytC). SPs represent a case of stable self-limited terminal assemblies made possible by the balance of attractive and repulsive forces between the building blocks that make them similar to other terminal assemblies. Applications of this research may include the realization of bionic assemblies with novel properties such as photoenzymatic activity [8] , [19] , [20] , enhanced stability [21] and potentially self-repair. Self-assembly of CdTe NPs and CytC Positively charged 3.8±0.4 nm CdTe NPs, stabilized by 2-(dimethylamino)ethanethiol (DMAET), are known to self-assemble into microscale sheets [3] , [22] . Among the wide range of choices for a ‘complementary’ biomolecule, we choose CytC, a well-studied protein 3.1 nm in size and a dipole moment as high as ~340 Debyes ( Supplementary Note 2 ) [23] , [24] . CytC alone does not reveal a tendency to self-assemble in aqueous solution at pH~7. The isoelectric point of CytC is 11.0; therefore, it is positively charged over a wide pH range. The choice of a positively charged protein for combining with positively charged NPs seems, at first glance, counterintuitive in promoting self-assembly. Conventionally, electrostatic attraction between oppositely charged building blocks drives self-assembly ( Supplementary Note 3 ) [9] , [12] , [25] . However, as we will demonstrate below, counterbalancing electrostatic repulsion with intermolecular attractive interactions including dipolar, hydrogen bonding, hydrophobic and van der Waals (vdW) forces is a viable approach that leads to terminal structures. Besides surfactants, self-limitation due to the counterbalance of attractive-repulsive forces was theoretically predicted [26] , [27] and observed for NPs [18] , [28] and electrified droplets of water. [29] Six micromolar NP dispersion at pH~5 is mixed with 6 μM CytC at pH~7. A stable NP-CytC dispersion with an electrokinetic potential (ζ) of +30 mV and pH~5.3 forms after ~48–72 h. The presence of CytC strongly affects the NP assembly pattern [3] . Examination by scanning electron microscopy (SEM) and transmission electron microscopy (TEM) reveals the formation of uniformly sized, spherical SPs with a TEM diameter of d TEM =94±5.6 nm ( Fig. 1a,e , and Supplementary Fig. 1 ) instead of large sheets typical of DMAET-CdTe NPs [3] . Their size distribution is narrow with a s.d. less than 7%. Dynamic light scattering (DLS) of 1:1 NP-CytC dispersion confirms the assembly of SPs with d DLS =99±19.0 nm ( Fig. 1f ), which matches the diameter determined from SEM/TEM data. The difference between d DLS and d TEM indicates incorporation of water molecules in the SPs, as is observed in many proteins and their assemblies [30] . We find that self-assembly into spheres is specific to the pairing of NPs and CytC in a 1:1 starting ratio. When NPs are the dominant components, there is an increasing tendency to form 2D structures ( Fig. 1b,c ). When proteins are dominant, the size distribution increased and large irregular aggregates appeared ( Fig. 1d , and Supplementary Fig. 2 ). Within them, 100-nm SPs are identifiable, indicating a specific tendency of CytC+DMAET-CdTe pairs to form spheres, unlike the diversity of other geometries observed before [2] , [3] , [4] , [21] . 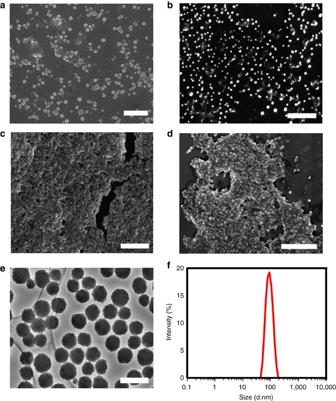Figure 1: Assembly of cadmium telluride nanoparticles(CdTe NPs) and cytochrome C (CytC). (a–d) Scanning electron miscroscopy (SEM) images of CdTe/CytC assemblies with molar ratio of CdTe:CytC as 1:1 (a), 2:1 (b), and 6:1 (c). 1:6 (d). (e) Transmission electron microscopy (TEM) image of CdTe/CytC supraparticles (SPs). (f) Size distribution of the self-assembled SPs by dynamic light scattering (DLS). Scale bar, 500 nm (a,c), 1 μm (b,d), and 200 nm (e). Figure 1: Assembly of cadmium telluride nanoparticles(CdTe NPs) and cytochrome C (CytC). ( a – d ) Scanning electron miscroscopy (SEM) images of CdTe/CytC assemblies with molar ratio of CdTe:CytC as 1:1 ( a ), 2:1 ( b ), and 6:1 ( c ). 1:6 ( d ). ( e ) Transmission electron microscopy (TEM) image of CdTe/CytC supraparticles (SPs). ( f ) Size distribution of the self-assembled SPs by dynamic light scattering (DLS). Scale bar, 500 nm ( a , c ), 1 μm ( b , d ), and 200 nm ( e ). Full size image The diameter of SPs shows limited dependence on the diameter of constitutive NPs. Specifically, a change in the NP average diameter from 2.7 nm to 7.2 nm results in a subtle change in diameter of SPs, remaining largely within experimental error ( Table 1 ). However, when the average diameter of NPs is increased to 13.5 nm, which is accompanied by a concomitant reduction in ζ, the average diameter of SPs increased markedly to 970 nm ( Table 1 and Supplementary Fig. 3 ). For most experiments, theoretical calculations and simulations reported here, we use the 3.8 nm of NPs. Table 1 Dependence of SP diameter on the NP diameter. Full size table We further examine the effect of ionic strength and temperature of assembly on the diameter of the SPs. The size of the SPs considerably decreases when the ionic strength of the assembly medium increases ( Fig. 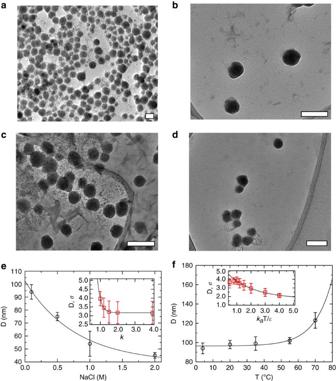Figure 2: Dependences of SP diameters on media parameters. (a–d) TEM images of SPs made in the solutions with (a) 0.1 M, (b) 0.5 M, (c) 1.0 M and (d) 2.0 M of NaCl. Scale bars are 100 nm. (e) Dependence of SP diameters on the NaCl concentration of NaCl and on inverse screening length in simulation (inset). (f) Temperature dependence of the SP diameters in experiment and in simulation (inset). The error bars in the experimental results (e,f) were obtained from the s.d. values from multiple experiments. Those in the simulation plots (insets ineandf) are the corresponding s.d. of the SP size distribution. 2a–d,e , Table 2 ). Meanwhile, the increase in temperature results in a slight increase in the SP average diameter ( Fig. 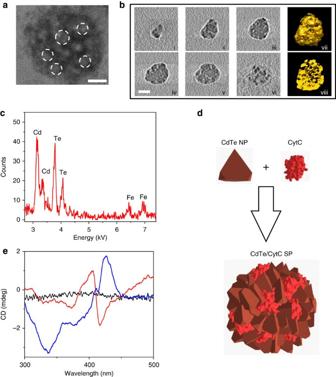Figure 3: Structural characterization of CdTe/CytC SPs. (a) High-resolution TEM (HR-TEM) image of the SP. Lighter areas correspond to CytC-rich phase (white-dashed circles), while the darker ones correspond to CdTe-rich phase. Scale bar, 10 nm. (b) TEM tomographic reconstructions of CdTe/CytC SP: X-Y slices (i-vi) of the SP, shown in every 4.8 nm through the volume. 3D surface rendering(vii) and cross-section (viii) of the SP (seeSupplementary Movie 1 and 2). Scale bar, 20 nm. (c) X-ray energy dispersive spectroscopy (XEDS) spectrum for an SP ina. (d) Schematics of the formation of CdTe-CytC SPs. (e) Circular dichroisum (CD) spectra for CytC (red, 6 μM), CdTe NPs (black, 6 μM), 1:1 mixture of CdTe/CytC after 72 (blue) h. 2f , Table 3 ). These trends indicate the possibility to control the dimension of CytC-CdTe assemblies; they also suggest that ‘phase diagrams’ of SP morphologies can be constructed based on these media parameters. Figure 2: Dependences of SP diameters on media parameters. ( a – d ) TEM images of SPs made in the solutions with ( a ) 0.1 M, ( b ) 0.5 M, ( c ) 1.0 M and ( d ) 2.0 M of NaCl. Scale bars are 100 nm. ( e ) Dependence of SP diameters on the NaCl concentration of NaCl and on inverse screening length in simulation (inset). ( f ) Temperature dependence of the SP diameters in experiment and in simulation (inset). The error bars in the experimental results ( e , f ) were obtained from the s.d. values from multiple experiments. Those in the simulation plots (insets in e and f ) are the corresponding s.d. of the SP size distribution. Full size image Table 2 Dependence of SP diameter on ionic strength. Full size table Table 3 Dependence of SP diameter on the temperature. Full size table The intermediate stages of the self-organization process indicate the path by which the SPs form. The appearance of particles with d DLS =126±9.7, 66±15.0, 72±9.4 and 100.6±17.3 nm are observed at 1, 24, 48 and 72 h, respectively ( Supplementary Fig. 4 ). This is accompanied by a gradual disappearance of signals with d DLS =5±0.4 and 20±1.4 nm, attributed to original NPs and early NP-CytC clusters, respectively. The initial increase and then decrease of d DLS values show that large aggregates with a broad size distribution form quickly, and subsequently condense and stabilize in size by 72 h. The sequence of the intermediate stages preceding the formation of stable SPs is confirmed by TEM images ( Supplementary Fig. 5 ). Supraparticle characterization High-resolution transmission electron microscopy (HRTEM) of the assemblies indicates that they consist of reticulated electron-transparent and electron-dense areas ( Fig. 3a , and Supplementary Fig. 6 ) with a characteristic size of ~5–7 nm. Tomographic 3D reconstruction images of the spherical SPs show that these areas interpenetrate each other ( Fig. 3b vii, viii, and Supplementary Movie 1 and 2 ) to form a network of tightly interconnected NP and CytC units. X-ray energy dispersive spectroscopy (XEDS) confirms the presence of both NPs and CytC ( Fig. 3c ). Individual NPs in semiconductor-rich areas can be distinguished by its crystal lattice with periodicity of 0.38 nm expected for CdTe (111) lattice planes ( Supplementary Fig. 6b ). We do not observe any specific order within the network, although the tight packing with volume density of NPs considerably higher than percolation threshold suggests it to be bi-continuous. Note that the interconnectivity of the NPs, which is essential for charge and exciton transfer within SPs, is likely to be non-random here and is governed by modified percolation theory applied to self-assembly [31] . Figure 3: Structural characterization of CdTe/CytC SPs. ( a ) High-resolution TEM (HR-TEM) image of the SP. Lighter areas correspond to CytC-rich phase (white-dashed circles), while the darker ones correspond to CdTe-rich phase. Scale bar, 10 nm. ( b ) TEM tomographic reconstructions of CdTe/CytC SP: X-Y slices (i-vi) of the SP, shown in every 4.8 nm through the volume. 3D surface rendering(vii) and cross-section (viii) of the SP (see Supplementary Movie 1 and 2 ). Scale bar, 20 nm. ( c ) X-ray energy dispersive spectroscopy (XEDS) spectrum for an SP in a . ( d ) Schematics of the formation of CdTe-CytC SPs. ( e ) Circular dichroisum (CD) spectra for CytC (red, 6 μM), CdTe NPs (black, 6 μM), 1:1 mixture of CdTe/CytC after 72 (blue) h. Full size image On the basis of the average volume of the SPs and the atomic ratio of Cd and Fe, the total number of CytC and NPs in a SP can be estimated to be 3.6 × 10 3 ±7.5 × 10 2 . The structures of individual SPs can be described by a schematic in Fig. 3d . We are interested in determining whether the process of SP formation ( Supplementary Figs 4 and 5 ) causes a significant degree of structural changes in the softer component, that is, CytC molecules, when it assembles with the more rigid components, that is, CdTe NPs. During SP assembly, the π-π* peak of CytC at 409 nm (Soret band) red-shifts to 415 nm, while the shoulder at 500 nm splits into two distinct peaks at 520 nm and 550 nm ( Supplementary Fig. 7a ). These transitions indicate a change in the oxidation state of the haem group in the protein from Fe +3 to Fe +2 upon SP assembly [32] ; from the extinction coefficient of the Fe +2 /Fe +3 at 550 nm, it is estimated that ~ 77% of the iron atoms are present in their reduced state in the assembled SPs ( Supplementary Note 4 ). After assembly with NPs, the proteins remain in a folded state; their denaturation would have manifested as a blue shift of the Soret band and disappearance of the peaks in 500–600 nm region, neither of which is observed in our system ( Supplementary Fig. 7a ). This conclusion is confirmed by essentially identical IR spectra of CytC before and after assembly with NPs ( Supplementary Fig. 8 ). The circular dichroism (CD) data further substantiate that CytC molecules incorporated in SPs retain their folded, although conformationally altered, state. Original CytC molecules have negative (−) CD peaks at 208 nm and 220 nm, corresponding to β-sheets and α-helices, respectively ( Supplementary Fig. 7d ). In the SPs, the positive CD peak representing α-helices at 225 nm dominates, and a new negative peak appears at 340 nm ( Fig. 3e and Supplementary Fig. 7d ). The conformational changes of CytC on interacting with NPs are also confirmed by examining the Soret region CD peaks that appear for free CytC at 408 nm (+) and 418 nm (−), typical of the haem group. The corresponding CD peaks in the assembled SPs become red-shifted and change signs ( Fig. 3e ), which correlates well with the change of the redox state of iron in the intact haem group. The dilution data in Supplementary Fig. 9 further confirm that these structural changes are intrinsic to SPs and are not due to intermediates or other macromolecular complexes. The observed changes in CD, UV spectra and the conformational transitions on assembly of CytC with NPs are reminiscent of those in CytC complexes with GroEL or Cytochrome C oxidase ( Supplementary Note 5 ) and those in concentrated solutions of globular proteins [26] . Assembly mechanism We now consider the mechanism of the formation of spherical monodisperse SPs. Since the components are similarly charged, we attribute their formation to a self-limiting process in which the electrostatic repulsion between the NPs and protein is overcome by weak attractive interactions, which corroborates previous findings ( Supplementary Discussion ) [18] . The overall attractive potential between the similarly charged CdTe NPs and CytC can be confirmed by calculations based on classical and extended Derjaguin, Landau, Verwey and Overbeek (DLVO) theory ( Fig. 4a , Supplementary Methods ). Although classical DLVO theory has multiple problematic points when applied to NPs, it is still instructive to show that the aggregation barrier in the pair potential is smaller than k B T . After addition of other terms, such as dipole–dipole, charge–dipole, and hydrophobic interactions (described in Supplementary Methods ) the pair potential becomes attractive for all separation distances. The non-monotonic nature of these interactions and their non-additivity at short separation distances are likely to further shift the balance towards the attractive interactions. Now the question is why such a pair potential does not lead to complete aggregation of the constituent particles. 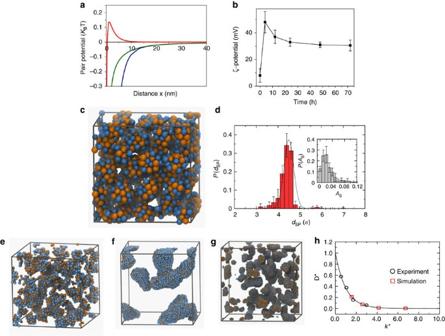Figure 4: Mechanism of self-assembly process. (a) Pair potential between CdTe NPs and CytC according to Derjaguin, Landau, Verwey and Overbeek (DLVO) and extended-DLVO (E-DLVO) theories:VDLVO(red);VE-DLVO1(green);VE-DLVO2(blue) (Supplementary Methods). (b) ζ-potential values for the assembly of CdTe NPs with CytC at different time intervals. Error bars indicate the s.d. values from multiple measurements. (c) Spherical assemblies formed by a mixture of 1,000 NPs (yellow) and 1,000 CytC units (blue) atρσ3=0.25. (d) Distribution of SP sizes and of the asphericity parameter (AS) (inset) of a system composed of 8,000 NPs and 8,000 CytC units (Supplementary Fig. 12a).AS=0 corresponds to perfect spheres. Error bars indicate 10 equilibrated, independent configurations separated by intervals of 2,000τ. (e,f) Snapshots of mixtures with NP/CytC molar ratios of 2:1 and 6:1, respectively. (g) A snapshot of a system identical to (c), but without the inter-SP charge-charge repulsion renormalization. The images in (c,e,fandg) were generated using the software VMD. (h) Experimental and simulated data fitted against decaying laws, that is f(x)~exp(−x), and plotted against dimensionless inverse screening length (κ*) and normalized diameters (D*) (seeSupplementary Methodsfor details). Figure 4: Mechanism of self-assembly process. ( a ) Pair potential between CdTe NPs and CytC according to Derjaguin, Landau, Verwey and Overbeek (DLVO) and extended-DLVO (E-DLVO) theories: V DLVO (red); V E - DLVO1 (green); V E - DLVO2 (blue) ( Supplementary Methods ). ( b ) ζ-potential values for the assembly of CdTe NPs with CytC at different time intervals. Error bars indicate the s.d. values from multiple measurements. ( c ) Spherical assemblies formed by a mixture of 1,000 NPs (yellow) and 1,000 CytC units (blue) at ρσ 3 =0.25. ( d ) Distribution of SP sizes and of the asphericity parameter ( A S ) (inset) of a system composed of 8,000 NPs and 8,000 CytC units ( Supplementary Fig. 12a ). A S =0 corresponds to perfect spheres. Error bars indicate 10 equilibrated, independent configurations separated by intervals of 2,000 τ . ( e , f ) Snapshots of mixtures with NP/CytC molar ratios of 2:1 and 6:1, respectively. ( g ) A snapshot of a system identical to ( c ), but without the inter-SP charge-charge repulsion renormalization. The images in ( c , e , f and g ) were generated using the software VMD. ( h ) Experimental and simulated data fitted against decaying laws, that is f(x)~exp(−x), and plotted against dimensionless inverse screening length ( κ *) and normalized diameters (D*) (see Supplementary Methods for details). Full size image Self-limiting processes, and therefore terminal assemblies, appear because the system evolves towards an equilibrium state as can be seen in the temporal profile of electrokinetic potential (ζ) during the assembly. Starting from ζ=+26 mV and +7 mV corresponding to individual CdTe NPs and CytC, respectively ( Supplementary Fig. 10 ), ζ rapidly increases from +8 mV (0 h) to +48 mV within the first 5 h. This state corresponds to the formation of large, dynamic, intermediate aggregates. Later, ζ reduces slightly to +37 mV (10 h) and plateaus at +31 mV (70 h, Fig. 4b ) due to the condensation of the intermediate aggregates. The ζ values match the trend of SP diameters that peak after ~1 h of the assembly time (see Supplementary Fig. 4 ). Computer simulations are performed to reveal further details of the self-limiting assembly of the SPs. On the basis of a coarse-grained model previously developed for CdTe NPs [3] ( Supplementary Fig. 11a ), the effective non-covalent interactions between NPs and CytC are described by the empirical 12-6 Lennard-Jones potential. The Yukawa potential models the screened charge–charge, dipole–dipole and dipole–charge interactions. As expected from previous studies, simulated tetrahedrally shaped DMAET-CdTe NPs self-assemble into flat sheets ( Supplementary Fig. 11b ) [3] . The presence of CytC markedly alters their assembly pathway to produce hybrid NP–protein SPs when the attraction of CytC to the NPs is sufficiently strong. ( Supplementary Fig. 11c ). To facilitate the computation while keeping essential physics of the self-limiting assembly process ( Supplementary Discussion ), we model NPs and proteins as spheres ( Fig. 4c–g ). Importantly, the inter-SP repulsion strength is renormalized as the assembly progresses ( Supplementary Discussion ) [27] , [33] , [34] so as to describe the structural adaptation of ionic clouds around NP and CytC during SP formation. We note that the SP–SP repulsion was renormalized in previous studies, for example, in refs 34 , 35 , presuming that the SPs already formed. This simplified model is useful to understand the control parameters for SP assembly and to demonstrate the generality of the assembly of NPs with proteins. Despite these simplifications, this model describes our experiments remarkably well. We observe the assembly of multiple SPs for a 1:1 molar ratio of the components, while deviations from this ratio produce assemblies with irregular shapes ( Fig. 4e,f ). Within the SPs, NPs and CytC form small clusters of a few particles ( Fig. 4c ) that correspond to domains ~6 nm in size, as observed from TEM ( Fig. 3a,b ). The simulated size distribution exhibits a pronounced peak ( Fig. 4d ) for the equilibrium state when the inter-SP repulsion balances the attraction between NPs and CytC. The small asphericity parameter ( Fig. 4d , inset) indicates that most of the simulated aggregates are indeed spherical. Multiple SPs at their terminal size do not coalesce because the repulsion from their constituents to any approaching NP or protein exceeds the net attraction ( Supplementary Fig. 12 ). The temporal profile of the potential energy plateaus for stable SPs, indicating the trend towards an equilibrium state ( Supplementary Fig. 12b ). We further observe that when the SPs reach their terminal size they become spherical in shape ( Supplementary Fig. 12c,d ). Continuous normalization of the charge screening conditions reflects the continuous change in the electric double layer for NPs as they assemble. When the inter-SP charge–charge repulsion renormalization is excluded from the simulation model, the assembly is not self-limiting, leading to infinite aggregation and non-uniform SPs ( Fig. 4g , and Supplementary Fig. 13 ) in disagreement with the experiments. This observation once again confirms that the assembly mechanism of terminal assemblies results from the balance between the net attractive forces between the NPs and CytC and their electrostatic repulsion, which should be renormalized with the SP sizes during aggregation. The effects of important media factors such as ionic strength and temperature on the size of the terminal SPs are also captured qualitatively in our simulation model. As the salt concentration is increased, the screening length of the electrostatic repulsion decreases, leading to the reduction in the effective repulsion between freely floating NPs and CytC. As a result, the number of NPs and CytC within the terminal SPs at the terminal size shifts to lower values given that the net attraction between individual units and the repulsion renormalization are unchanged. The decrease in the SP terminal size with the increased NaCl concentration ( Fig. 2e ) is also qualitatively recovered in our simulation model ( Fig. 2e , inset). The agreement between experimental and simulation data is pronounced when we fit the two data sets with decaying laws and plot them using dimensionless axes ( Fig. 4h , Supplementary Methods ). Meanwhile, the temperature dependence of the SP terminal size is consistent with experimental data in the lower temperature regime where k B T / ε ~1.0 ( Fig. 2f ) with epsilon being the well depth of the Lennard-Jones potential. In this temperature range, the net effective attraction between NPs and CytC is comparable to thermal fluctuations, and the terminal SP size is fairly insensitive to temperature. For k B T / ε much greater than 1.0, the attraction strength becomes weaker than thermal fluctuations, and the simulation results diverge from experimental observation with the decrease in the SP terminal size ( Fig. 2g , inset). This divergence can be attributed to the CytC molecules adopting conformations other than the folded state being used in the current model. Photoenzymatic activity Terminal assemblies enable a simple means for fabricating complex bio-nano systems from a variety of components. They can also be called ‘bionic’ assemblies because they combine the properties of inorganic and biological components. A new redox enzyme, namely nitrate reductase (NRed), is incorporated as an additional component in SPs as they assemble from CytC and NPs. NRed integration into SPs leads to an increase in SP size and decrease in ζ-potential while maintaining SP sphericity ( Supplementary Figs 15a,b and 16). Various spectroscopy data indicated that 25±8 NRed molecules are incorporated in each SPs; this number correlates well with the observed increase in SP diameter ( Supplementary Fig. 15b–e ). The positions of all peaks in the UV-Vis/CD spectra remain unchanged, indicating that the electronic state and conformation of the CytC molecules in the SPs are preserved ( Supplementary Fig. 15f,g ). Nicotinamide adenine dinucleotide phosphate, (NADPH), which serves as a sacrificial electron donor, is added to the SP dispersion. Incorporation of NADPH in the SPs is observed based on XEDS data ( Supplementary Fig. 15h ). Direct reduction of NO 3 − by NADPH cannot occur and must have been catalysed by NRed. We examine whether this catalytic process can be driven by light adsorption into CdTe. The direct electron transfer from CdTe to NRed; it is slow and has to be mediated by CytC. The rate of NO 2 − production by SP-NRed in presence of NADPH increased fourfold when we illuminated the SPs at 470 nm—the absorption peak of CdTe NPs ( Fig. 5a ). This indicates that the sequence of electron transfer reactions NADPH→CdTe ( hν )→ CytC→NRed→NO 3 − is likely to occur. The reduced form of CytC present in SPs ( Fig. 3 ) can initiate the process of NO 3 − conversion. Subsequently the photo-excited electrons from CdTe NPs are continuously supplied to CytC, which shuttles them to NRed. The holes in CdTe are scavenged by NADPH ( Supplementary Note 6 ). Dense packing of all the organic and inorganic building blocks within SPs and the large interfacial area of the bicontinuous percolated structure of SPs facilitate all the electron transfer reactions. The importance of dense packing could also be seen for clusters of inorganic catalysts [36] . Side reactions, such as reduction of NP holes by oxidizable residues on the proteins, for example, tyrosine, in CytC, are nevertheless highly probable, similarly to bioconjugates [19] , [36] , [37] . 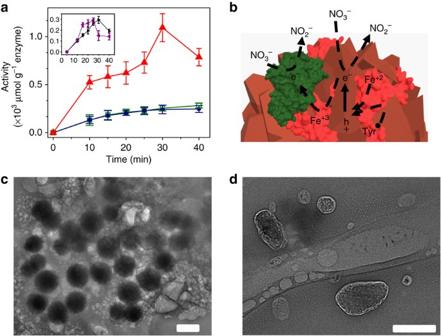Figure 5: Functional integration of SPs with photoenzymatic activity. (a) Formation of nitrite for SP-nicotinamide adenine dinucleotide phosphate (NADPH)-nitrate reductase (NRed) (red) excited at 470 nm and for NADPH-NRed (green) and SP-NADPH-NRed in dark (blue). Inset: formation of nitrite for NADPH-NRed being excited at 470 nm in presence of only one of SP components: either CdTe NPs (black) or CytC (purple) when no hybrid SPs were formed. Errors bars are based on triplicate experimental measurements. (b) Schematics of the reactions on the photoexcitation of SP-NADPH-NRed. Nitrate reductase is represented as a surface model from PyMol software, PDB entry is 2BIH. TEM images of (c) SP-NADPH-NRed after 20 min and (d) after 40 min of the photoenzymatic reaction. Scale bar, 100 nm. Figure 5: Functional integration of SPs with photoenzymatic activity. ( a ) Formation of nitrite for SP-nicotinamide adenine dinucleotide phosphate (NADPH)-nitrate reductase (NRed) (red) excited at 470 nm and for NADPH-NRed (green) and SP-NADPH-NRed in dark (blue). Inset: formation of nitrite for NADPH-NRed being excited at 470 nm in presence of only one of SP components: either CdTe NPs (black) or CytC (purple) when no hybrid SPs were formed. Errors bars are based on triplicate experimental measurements. ( b ) Schematics of the reactions on the photoexcitation of SP-NADPH-NRed. Nitrate reductase is represented as a surface model from PyMol software, PDB entry is 2BIH. TEM images of ( c ) SP-NADPH-NRed after 20 min and ( d ) after 40 min of the photoenzymatic reaction. Scale bar, 100 nm. Full size image In the absence of light, the presence of the SPs has virtually no effect on the activity of the enzyme ( Fig. 5a ). Control experiments confirm the significance of the NPs and SPs for the photoenzymatic NO 3 − reduction. These include the enzyme reaction (i) either with CdTe NPs or (ii) with CytC upon illumination ( Fig. 5a , inset). None of the control experiments shows enzyme activity as high as for the illuminated SP-NRed in the presence of NADPH. The assembled SPs remain intact after 20 min of photoreaction. However, the disassembly of SP-NRed occurred after ~30 min of SP-NRed’s exposure to light ( Fig. 5c,d ), which was synchronized with the drop in photoenzymatic activity ( Fig. 5a , Supplementary Fig. 17 ). The decrease in enzymatic activity is attributed to irreversible oxidation of the NPs by the photogenerated holes. This results in removal of DMAET ligands from the surface of the NPs, and therefore the loss of attractive intermolecular interactions. The synchronization of the drop in enzymatic reduction and onset of disassembly vividly demonstrates that the formation of the terminal SPs is necessary to obtain higher photoenzymatic activity. TEM images of SPs after extended photoreaction support this conclusion ( Fig. 5d ). In summary, CdTe NPs and like-charged proteins self-organize into self-limiting SPs, following a pattern previously unseen for the individual components. These terminal superstructures display complex internal organization and can incorporate multiple biological components. We also demonstrate that the protein component retains its functionality. ‘Bionic’ integration of the light absorbing properties of the NPs and the catalytic properties of the enzyme was achieved. Since only generic attractive-repulsive forces are required for formation of the terminal SPs, we expect that they can be made from a large variety of NPs and proteins. The simplicity of their preparation is conducive to a large variety of such structures that can form in the laboratory and in nature. We stress that this simplicity of preparation and seemingly good match with theoretical and computational description of the attraction-repulsion balance do not imply the simplicity of the interactions between CdTe and CytC as well as other proteins/NPs. The altered conformation of the protein is a clear indication of their complexity and non-monotonic nature of such interactions associated with the ‘softness’ of the interacting particles. Consideration of these details in subsequent theoretical and computational treatments will allow provide prediction of explicit NP interaction and effective integration of inorganic and biocatalytic properties in SP assemblies. Synthesis of DMAET-stabilized CdTe NPs DMAET-CdTe NPs were prepared following the previous study [22] . In brief, ~0.7 g of Cd(ClO 4 ) 2 ·6H 2 O (Alfa Aesar) dissolved in 200 ml of water was mixed with ~0.45 g of DMAET (Sigma-Aldrich). Subsequently, pH of the medium was adjusted to be ~5.5 by addition of 0.1 M HCl solution. The reaction mixture was placed in three 250 ml neck round bottom flask with a septum, valve and condenser, and was bubbled with N 2 gas for at least 30 min. H 2 Te gas formed by reacting~0.2 g of Al 2 Te 3 (Materion) with 0.5 M-H 2 SO 4 was passed through the reaction mixture for 10 min at room temperature. Then, the reaction proceeded for 1–1.5 h under magnetic stirring at 100 °C. The reaction was stopped by cooling down the reactor at room temperature for ~30 min. The average diameter of the synthesized NPs was 3.8±0.4 nm. The reaction time varied to obtain different sizes of the NPs. Assembly of CdTe/CytC SPs Typically, 1 ml of NP dispersion containing 6 μM of NPs was precipitated at 4 °C for 24 h. Subsequently, the dispersion was centrifuged at 6,000 r.p.m. for 20 min at 15 °C. The supernatant was discarded, and the NPs were redispersed in 1 ml of water at pH 5 (adjusted by the addition of 0.1 M HCl). Finally, the NP dispersion was mixed with 20 μl of 300 μM-CytC aqueous solution and was stored for 72 h. The assembly medium contained desired concentrations (0.1, 0.5, 1.0, 2.0 M) of NaCl, or it was stored at different temperatures (4, 20, 35, 55, 70 °C). Typically, samples for TEM/SEM studies were diluted before imaging. Enzymatic reduction of nitrate Ten microlitres of enzyme, NRed, solution (Cayman Chemical) was added to 770 μl of aqueous solution containing CdTe/CytC SP (40 μl), cofactor (NADPH, 10 μl, Cayman Chemical) and NaNO 3 (150 μl, 200 mM). The solution was placed in in 800 μl quartz cuvette (Starna cells) and illuminated at 470 nm via Horiba FluoroMax-3 monochromator for 1 h with slit width for excitation at 20 nm. The wavelength matched to the onset of excitonic absorption of CdTe NPs in the bionic SPs. During illumination, 30 μl of aliquots diluted with 470 μl of water at desired time intervals were taken for analysis. Nitrate reduction assay Before the assay, each of 500 μl of diluted samples was mixed with 50 μl of 2,3-diaminonaphthalene (DAN) and 100 μl of 2.8 M-NaOH solution (Cayman Chemical). Fluorescence emission at 417 nm of the samples was recorded by exciting the samples at 375 nm (Synergy2 plate reader, Biotek). The activity was measured by a standard fluorescence assay method to quantify produced NO 2 − (μmol g −1 -enzyme) ( https://www.caymanchem.com/pdfs/780051.pdf. ). The concentration of NO 2 − was determined by a standard plot of different concentrations of NO 2 − (see Supplementary Fig 18 ). How to cite this article: Park, J. I. et al. Terminal supraparticle assemblies from similarly charged protein molecules and nanoparticles. Nat. Commun. 5:3593 doi: 10.1038/ncomms4593 (2014).